Interfacial liquid-state surface-enhanced Raman spectroscopy Oriented assemblies of functional nanoparticles, with the aid of external physical and chemical driving forces, have been prepared on two-dimensional solid substrates. It is challengeable, however, to achieve three-dimensional assembly directly in solution, owing to thermal fluctuations and free diffusion. Here we describe the self-orientation of gold nanorods at an immiscible liquid interface (that is, oleic acid–water) and exploit this novel phenomenon to create a substrate-free interfacial liquid-state surface-enhanced Raman spectroscopy. Dark-field imaging and Raman scattering results reveal that gold nanorods spontaneously adopt a vertical orientation at an oleic acid–water interface in a stable trapping mode, which is in good agreement with simulation results. The spontaneous vertical alignment of gold nanorods at the interface allows one to accomplish significant additional amplification of the Raman signal, which is up to three to four orders of magnitude higher than that from a solution of randomly oriented gold nanorods. Oriented assemblies of functional colloidal nanoparticles [1] , [2] , [3] , [4] , [5] , [6] , [7] , [8] , [9] , [10] , [11] , [12] , [13] , [14] , [15] , [16] , [17] , [18] , [19] , [20] are important for both fundamental science and technological applications. Such assemblies have been realized on two-dimensional (2D) solid substrates by utilizing evaporation-based convection [6] , [7] , capillary interaction [8] , electric fields [9] , [10] , substrate templating [11] , [12] and surface tailoring of nanoparticles [13] , [14] . However, robust control over the orientation and position of nanoparticles in 3D solutions remains a formidable challenge, owing to thermal fluctuations and diffusion. Such a capability could allow for a new route to the formation of functional materials, as well as the development of new types of platforms, for molecular detection and soft-matter characterization. Herein, we demonstrate that an oleic acid–water interface in the absence of external fields and additional programmable molecules can orient gold nanorods (GNRs) in order to minimize an interfacial energy. We exploit this novel phenomenon to subsequently present simple and versatile substrate-free liquid-state surface-enhanced Raman spectroscopy. The collective and vertical orientation of GNRs in a stable trapping mode is directly visualized by dark-field microscope. Analytical and numerical calculations also support that GNRs randomly oriented in an aqueous solution vertically align at the oil–water interface following the addition of oleic acid. To further verify our experimental observations and calculations, as well as demonstrate our interfacial liquid-state label-free sensing technique, Raman scattering experiments are carried out. It is expected that such uniform orientation of the GNRs at the interface should result in the dramatic additional enhancement of surface-enhanced Raman scattering (SERS) signals when compared with the signals measured directly from a solution of randomly oriented GNRs. Our technique has several key benefits: it is simple and fast as it involves mixing an aqueous GNR solution with targets of interest, adding oleic acid, illuminating the clearly visible interface between the two immiscible liquids with laser and collecting fingerprint information; the chemicals (including GNRs) and equipment (a portable Raman spectrometer) required are readily available; it can provide a platform for high-throughput screening of targets, which may create new opportunities for SERS applications; by taking advantage of the spontaneous vertical alignment of the GNRs, we can obtain a significant additional signal enhancement factor (EF) of up to 10 4 ; and, finally, self-oriented GNRs at the interface allow for the detection of both oil-soluble and water-soluble molecules. Our versatile interfacial label-free detection technique therefore has great potential in the precise characterization of soft matters. Vertical orientation of GNRs at oleic acid–water interface Our proposed method that is based on the vertical orientation of GNRs at the interface is illustrated in Fig. 1 ( Supplementary Movie 1 ). In order to obtain the direct evidence for such orientation, we performed dark-field imaging with designing a fluidic chamber ( Fig. 2a ). Supplementary Movie 2 and its time-resolved snapshots ( Fig. 2b ) show that GNR (left spot) moves randomly in water (near the interface); however, once the GNR reaches at the oleic acid–water interface, it does not move owing to stable trapping mode (that is, the lowest-energy level). In principle, polarization-dependent dark-field microscopy provides us the direct evidence of the vertical orientation of GNRs. If GNR is vertically oriented at the liquid–liquid interface, we would expect an identical scattering imaging regardless of the polarization of incident light owing to a symmetrical orientation whereas non-vertically oriented GNRs would show a polarization-dependent scattering owing to an asymmetric orientation with respect to the incident polarization light ( Fig. 2a ). Figure 2c show the dark-field scattering images of GNRs for different linear polarization of incident light. 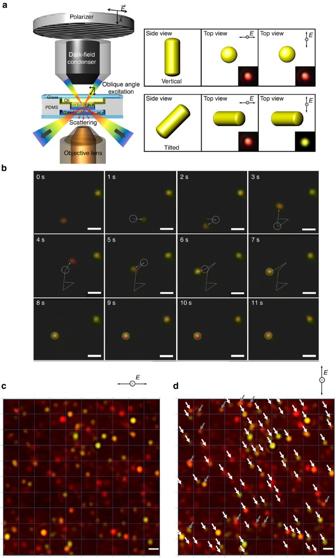Figure 2: Vertical orientation of GNRs at the oleic acid–water interface. (a) Dark-field imaging setup with a special fluidic chamber and conceptual polarization-dependent scattering colours in accordance with the orientation of GNR. (b) Time-resolved snapshots showing interfacial trapping of the GNR captured from theSupplementary Movie 2. All images for the interface are from top view. The right spot indicates the GNR being trapped earlier than recording. (c,d) Dark-field scattering images of GNRs for different linear polarization of incident light. Based on the observation of the GNRs in the stable trapping mode at the interface, only motionless spots are considered. Note that we did not take spots being far from the focal plane, or moving to other positions, or newly appearing into consideration when comparing the two images obtained from different polarization. Scale bar, 1 μm. Note that only motionless spots in the two images are considered. White arrows indicate that most of the spots at the interface (77 among 89 spots, see also Supplementary Fig. S1 ) show nearly identical scattering colour for both polarizations while only a small number of the spots indicated by grey arrows accompany the change in the scattering colour. This result directly suggests that the GNRs are likely to adopt the vertical orientation at the interface. Note that the variation in the initial scattering colour (from yellow and orange, to red) can be mainly attributed to the aspect ratio distribution of the GNRs we prepared (from 2 to 6, Supplementary Fig. 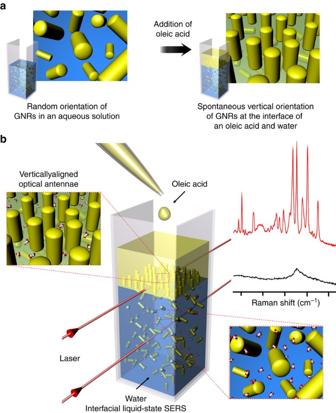S2 ). Figure 1: Schematic illustration of substrate-free interfacial liquid-state SERS. (a) Spontaneous and collective vertical alignment of GNRs (GNRs) at the oleic acid–water interface. (b) Interfacial liquid-state label-free detection method consists of three steps including mixing GNRs and targets, and adding oleic acid, followed by Raman measurement at the clearly visible interface. Figure 1: Schematic illustration of substrate-free interfacial liquid-state SERS. ( a ) Spontaneous and collective vertical alignment of GNRs (GNRs) at the oleic acid–water interface. ( b ) Interfacial liquid-state label-free detection method consists of three steps including mixing GNRs and targets, and adding oleic acid, followed by Raman measurement at the clearly visible interface. Full size image Figure 2: Vertical orientation of GNRs at the oleic acid–water interface. ( a ) Dark-field imaging setup with a special fluidic chamber and conceptual polarization-dependent scattering colours in accordance with the orientation of GNR. ( b ) Time-resolved snapshots showing interfacial trapping of the GNR captured from the Supplementary Movie 2 . All images for the interface are from top view. The right spot indicates the GNR being trapped earlier than recording. ( c , d ) Dark-field scattering images of GNRs for different linear polarization of incident light. Based on the observation of the GNRs in the stable trapping mode at the interface, only motionless spots are considered. Note that we did not take spots being far from the focal plane, or moving to other positions, or newly appearing into consideration when comparing the two images obtained from different polarization. Scale bar, 1 μm. Full size image Theoretical calculation of GNR orientation at interfaces To further elaborate the vertical orientation of the GNRs at the interface, we calculate the interfacial energy to determine the equilibrium orientation of interface-trapped GNRs. The aspect ratio of the GNR in the calculation is set to 3.7, which corresponds to the average aspect ratio of the GNRs used in the experiment ( Supplementary Fig. S2 ). We analytically calculated the surface area of the GNR in contact with each fluid phase and the interfacial area occupied by the particle. The calculated area and the corresponding interfacial tensions are used to numerically determine the interfacial energy, which is a function of orientation angle and vertical displacement with respect to the interface (see Supplementary Note 1 ) as described by equation (1). Note that thermal fluctuation, charge effect, interparticle interaction and gravitational force can be neglected owing to: the size of the GNR [21] , [22] , the interparticle distance and the fact that the pH value of the GNR solution is similar to the p K a of oleic acid, respectively. In equation (1), m represents a fluid medium such as air, water and oleic acid. and are the areas of the ends (top and bottom) and the side of the GNR contacting each medium, respectively. and correspond to the interfacial tension of the contacted surface area of the GNR with each medium. is the interfacial tension between the two fluids. A represents the interface area occupied by the particle ( Supplementary Fig. S3 ). For a given orientation of the GNR at the interface, the surface of the GNR can be divided into four regions, as described in Fig. 3a and Supplementary Fig. S3 . As the GNR is stabilized by cetyltrimethylammonium bromide (CTAB) [23] , [24] , which preferentially binds to the side surface rather than both ends owing to the size of its head group [25] , the local density of CTAB on the side is assumed to be much greater than that on the ends. Although the number of CTAB layers on the GNR surface may differ in water and oleic acid, it is assumed that this has a negligible effect on the interfacial tension. Given the aforementioned considerations, the interfacial tensions are determined using reported values [26] , [27] and our own estimation ( Supplementary Note 2 ). 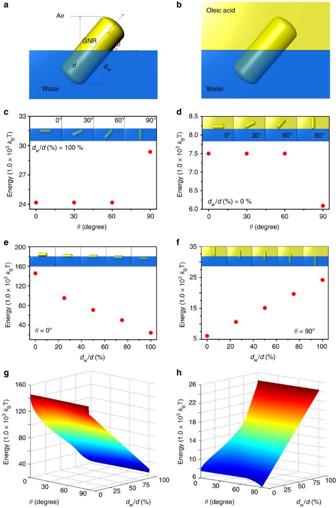Figure 3: Theoretical calculation of GNR orientation at interfaces. (a,b) Calculation parameters:θis the angle formed between the long axis of the GNR and the interface,drepresents the distance from the bottom to the top of the GNR anddwis the distance from the bottom of the GNRs to the air–water interface (a) and the oleic acid–water interface (b). (c,d) Plots depicting the calculated interfacial energy as a function ofθat fixed positions corresponding todw/d=100% at the air–water interface (c) and 0% at the oleic acid–water interface (d). (e,f) Interfacial energy profiles as a function ofdw/dwithθfixed to a value of 0° at the air–water interface (e) and 90° at the oleic acid–water interface (f). (g,h) Calculated interfacial energy profiles with respect to orientation angle (θ) and vertical displacement (dw/d) at the air–water interface (g) and the oleic acid–water interface (h).kBTcorresponds to the available thermal energy. Figure 3: Theoretical calculation of GNR orientation at interfaces. ( a , b ) Calculation parameters: θ is the angle formed between the long axis of the GNR and the interface, d represents the distance from the bottom to the top of the GNR and d w is the distance from the bottom of the GNRs to the air–water interface ( a ) and the oleic acid–water interface ( b ). ( c , d ) Plots depicting the calculated interfacial energy as a function of θ at fixed positions corresponding to d w /d =100% at the air–water interface ( c ) and 0% at the oleic acid–water interface ( d ). ( e , f ) Interfacial energy profiles as a function of d w /d with θ fixed to a value of 0° at the air–water interface ( e ) and 90° at the oleic acid–water interface ( f ). ( g , h ) Calculated interfacial energy profiles with respect to orientation angle ( θ ) and vertical displacement ( d w /d ) at the air–water interface ( g ) and the oleic acid–water interface ( h ). k B T corresponds to the available thermal energy. Full size image Figure 3c include plots of the typical calculated interfacial energy as a function of orientation angle ( θ ) with a fixed vertical displacement of d w /d =100% for the air–water interface ( Fig. 3c ) and 0% for the oleic acid–water interface ( Fig. 3d ). At the air–water interface, GNR possesses the largest interfacial energy when vertically oriented (90°) while GNRs with other orientation angles show smaller and identical interfacial energies. On the contrary, at the oleic acid–water interface, the interfacial energy at an orientation angle of 90° is smaller than those at other orientation angles by ~1,500 k B T . The magnitude of the energy barrier between the vertical and horizontal orientations is large enough that a transition between the two orientations driven by thermal fluctuation ( k B T ) is unlikely to occur. In addition, at the air–water interface, when θ is fixed to a value of 0°, the energy decreases as the GNR is gradually immersed in the water layer ( Fig. 3e ). At the oleic acid–water interface, the energy gradually decreases as the GNR with a fixed orientation angle of 90° rises into the oleic acid layer ( Fig. 3f ). The equilibrium energy minima as a function of orientation angle and vertical displacement are represented on the 3D contour surface shown in Fig. 3g (and Supplementary Fig. S4 ). The global energy minimum for the GNR at the oleic acid–water interface occurs at an orientation angle of 90°, indicating that the GNRs prefer to adopt a single orientation and a vertical displacement of 0% ( Fig. 3h ). On the other hand, GNRs at the air–water interface possess a minimum energy when submerged in water with no preferred orientation ( Fig. 3g ). Interfacial liquid-state SERS technique We next carried out the measurement of Raman scattering under an excitation of 785 nm laser ( Supplementary Fig. S5 ). The merits of the Raman experiments in our study are twofold: it provides further experimental verification of the vertical orientation of GNRs at the interface, and is the first demonstration of the substrate-free interfacial liquid-state surface-enhanced Raman spectroscopy. In principle, the orientation of anisotropic gold nanoparticles (for example, dimers [18] and GNRs [28] ) can be indirectly resolved by Raman scattering experiments. In our experiment, GNRs with a longitudinal plasmon resonance of ~785 nm were used ( Supplementary Fig. S2 ). Because of the anisotropic structure of the GNRs, two plasmon resonance bands are induced by the transverse and longitudinal oscillations of free electrons [29] . Note that the SERS intensities depend strongly on both the orientation of the GNRs and the illumination direction of the laser [18] , [28] , [30] . When the long axis of the GNRs is perpendicular to the illumination direction of the incident light, a resonance condition in a far-field regime is satisfied resulting in significant amplification of the Raman signal ( Fig. 4d and Supplementary Fig. S6a ). On the other hand, if the long axis of the GNRs is aligned parallel to the illumination direction, no Raman enhancement would occur ( Fig. 4e and Supplementary Fig. S6b ). It is important to note that all SERS data are collected within 20 s of the addition of oleic acid in order to neglect the effects of diffusion (for example, diffusion of target molecules [31] and GNRs [32] to the interface) on the measurements. 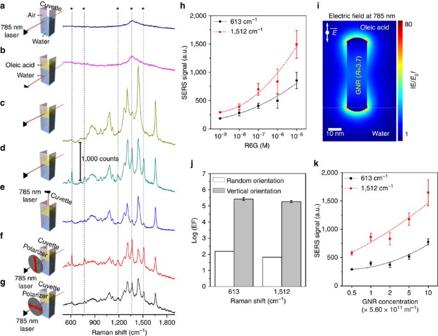Figure 4: Interfacial liquid-state SERS with vertical orientation of the GNRs. (a–g) Raman spectra measured at the air–water interface (a), in the water layer (b), in the oleic acid layer (c) and at the oleic acid–water interface (d–g). Positions marked with an asterisk correspond to representative Raman peaks of R6G (Supplementary Fig. S7). The SERS signals of R6G are collected at the oleic acid–water interface under four different laser illumination conditions (d, horizontal illumination to the interface;e, perpendicular illumination;f, horizontal illumination of a perpendicularly polarized laser; andg, horizontal illumination of a horizontally polarized laser). (h) Concentration-dependent intensity changes at two indicator peaks (that is, 613 and 1,512 cm−1) of R6G. SERS measurement was performed with varying concentrations over several orders of magnitude (from 1 nM to 10 μM). (i) Simulated electric field distribution of a single GNR (aspect ratio=3.7) under 785-nm laser excitation. The intensity scale is normalized asE/E0. (j) Comparison of Raman EF measured from vertically oriented GNRs at the interface with EF measured from the randomly oriented GNR in a solution. (k) Effect of the preconcentration of GNRs on the SERS signal at the interface for 1 μM R6G solutions. The preconcentration factor is the dilution or concentration ratio based on the initial concentration of the as-made GNRs. All experiments were repeated five times. Each error bar indicates the s.d. Figure 4: Interfacial liquid-state SERS with vertical orientation of the GNRs. ( a – g ) Raman spectra measured at the air–water interface ( a ), in the water layer ( b ), in the oleic acid layer ( c ) and at the oleic acid–water interface ( d – g ). Positions marked with an asterisk correspond to representative Raman peaks of R6G ( Supplementary Fig. S7 ). The SERS signals of R6G are collected at the oleic acid–water interface under four different laser illumination conditions ( d , horizontal illumination to the interface; e , perpendicular illumination; f , horizontal illumination of a perpendicularly polarized laser; and g , horizontal illumination of a horizontally polarized laser). ( h ) Concentration-dependent intensity changes at two indicator peaks (that is, 613 and 1,512 cm −1 ) of R6G. SERS measurement was performed with varying concentrations over several orders of magnitude (from 1 nM to 10 μM). ( i ) Simulated electric field distribution of a single GNR (aspect ratio=3.7) under 785-nm laser excitation. The intensity scale is normalized as E / E 0 . ( j ) Comparison of Raman EF measured from vertically oriented GNRs at the interface with EF measured from the randomly oriented GNR in a solution. ( k ) Effect of the preconcentration of GNRs on the SERS signal at the interface for 1 μM R6G solutions. The preconcentration factor is the dilution or concentration ratio based on the initial concentration of the as-made GNRs. All experiments were repeated five times. Each error bar indicates the s.d. Full size image The SERS intensities of 1 μM aqueous solutions of rhodamine 6G (R6G) were measured as a function of the direction and polarization of the laser light as well as illumination position ( Fig. 4a–g ). The intrinsic Raman transitions of R6G were observed at 613, 770, 1,182, 1,317, 1,365 and 1,519 cm −1 ( Supplementary Fig. S7 ). In SERS measurements, we monitored only the peaks at 613 and 1,512 cm −1 as the other transitions overlap those of oleic acid ( Supplementary Fig. S8 ). The slight shift in peak position (1,519 to 1,512 cm −1 for R6G) between the normal Raman measurement and the SERS measurement is commonly observable [33] , [34] , [35] . When the air–water interface ( Fig. 4a ) and the water layer ( Fig. 4b ) containing GNRs was illuminated with 785-nm laser light, no R6G Raman signal was observed. Following the addition of oleic acid, Raman transitions of oleic acid (1,085, 1,306, 1,443 and 1,657 cm −1 , see Supplementary Fig. S8 ) were observed upon illumination to the oleic acid layer, as expected ( Fig. 4c ). Interestingly, it is only at the interface between oleic acid and water that Raman signals of both R6G and oleic acid were clearly observed ( Fig. 4d–g , Supplementary Fig. S9 and Supplementary Movie 1 ). We further examined the peak intensities of R6G by varying the illumination direction. The strongest intensity was obtained from the interface under horizontal illumination ( Fig. 4d and Supplementary Fig. S6a ). Figure 4e shows the SERS spectrum under perpendicular illumination to the interface ( Supplementary Fig. S6b ). The intensities were decreased to 15% of those obtained under horizontal illumination ( Fig. 4d ). In addition, the peak intensities displayed a strong dependence on the polarization angle of the illumination source, which is depicted by the arrows in Fig. 4f . When the laser source is perpendicularly polarized to the interface (that is, the polarization along the long axis of GNR, Supplementary Fig. S6c ), the SERS intensity increases by a factor of 3 over the intensities measured under horizontal polarization ( Supplementary Fig. S6d ). Taken together, the Raman scattering measurements also confirm the preferential assembly of vertically oriented GNRs at the oil–water interface. Having experimentally shown that a vertical orientation is the preferred orientation adopted by the GNRs at the oleic acid–water interface, we sought to evaluate the sensing performance of our technique. For determining the limit of detection, the concentrations of R6G were varied by an order of magnitude over a range of 1 nM to 10 μM. Note that the intensities of the Raman peaks attributed to oleic acid at the interface over the range of R6G concentrations examined were nearly identical. As shown in Fig. 4h , by monitoring the intensities of two indicator peaks (613 and 1,512 cm −1 ), the limit of detection of the method was found to be between 1 and 10 nM. Considering the charge and constituent atoms of R6G, the observed SERS signal can be mainly attributed to R6G molecules in very close proximity to the GNRs. The simulation of the local field enhancement ( E / E 0 ) under 785 nm excitation ( Fig. 4i ) shows that the electric field is strongly enhanced around the end surface of the vertically oriented GNR. It is important to address the magnitude of SERS enhancement attributed to the vertically oriented GNRs at the interface. We estimated EFs according to the equation, EF=( I SERS / C SERS )/( I RS / C RS ), where I SERS and I RS represent the measured SERS signal and Raman signal, and C is the concentration of R6G. Raman signals of R6G measured in solution containing randomly oriented GNRs are not detectable below concentrations of 10 μM. Considering that no Raman signal of R6G in the absence of GNRs is detectable either in solution or at the interface below concentrations of 1 mM, Raman EFs from vertically oriented and randomly oriented GNR systems can be estimated to be ~10 6 –10 5 and 10 2 ( Fig. 4j ), respectively. Consequently, the additional SERS EF stemming purely from the vertical orientation of the GNRs lies between 10 4 and 10 3 . It is noteworthy that, even under the same concentration of 10 μM, Raman counts from the vertically oriented GNRs (that is, from the oleic acid–water interface) is ca. 120 times higher than those from the randomly oriented GNRs (that is, from a solution). It is clear that the number of GNRs at the interface can be increased with increasing a GNR concentration. To evaluate the dependence of our interfacial liquid-state SERS technique on the GNR concentration ( Fig. 4k ), the intensities of the R6G peaks were measured as a function of the GNR concentration. The concentration of R6G was fixed at 1 μM in each case. As expected, the SERS signal gradually increases as the GNR concentration increases. When the concentration of GNRs is increased to ten times (by centrifugation) greater than the value obtained from the typical synthetic protocol [23] , the intensity increased by a factor of two. As the calculated interparticle distance (~880 nm at 5.6 × 10 11 ml −1 and 270 nm at 5.6 × 10 12 ml −1 ) and the surface charge of the GNR allow us to rule out any plasmonic coupling between GNRs (that is, keeping the electric field enhancement per GNR constant), it is understandable that the increase of GNR concentration under the same R6G concentration results in the monotonous increase of the number of molecules near GNRs. Note that no aggregation is observed throughout our experiments ( Supplementary Fig. S10 ). The effect of GNR length on the signal intensity was examined by additional simulation and Raman measurements by using longer GNRs with aspect ratios of 13 ( Supplementary Fig. S11 ) and 18. Simulation results suggest that longer GNRs maintain the vertical orientation at the oleic acid–water interface ( Supplementary Fig. S12 ). However, no Raman peaks corresponding to R6G are observed in the cases of longer GNRs ( Supplementary Fig. S13 ), which is probably owing to the non-matching of the longitudinal plasmon wavelength of GNR with 785 nm laser. For the reproducibility, the SERS signals measured from 15 samples prepared by the same protocol are almost the identical, indicating the high uniformity and repeatability of our interfacial SERS technique ( Supplementary Fig. S14 ). Versatility of our interfacial liquid-state SERS technique To further validate our technique, other molecules, including water-soluble 1-1′-diethyl-2-2′-cyanine iodide (DCI) and oil-soluble 1,2-bis(4-pyridyl)ethane (BPE), were tested ( Fig. 5 ). Before measuring their respective SERS response, a Raman spectrum of each molecule was collected for reference ( Supplementary Fig. S15 ). For DCI, Raman transitions were detectable at 609 and 1,389 cm −1 above concentrations of 10 nM at the oleic acid–water interface ( Fig. 5a and Supplementary Fig. S16 ). In a solution containing randomly oriented GNRs, no DCI Raman signal was detectable below a concentration 100 μM (data not shown) and thus, the additional EF is found to be ~10 4 . Similarly for oil-soluble BPE, appreciable SERS signals at 1,200 and 1,639 cm −1 were observed ( Fig. 5b ) at the oleic acid–water interface. However, no remarkable BPE Raman signals could be detected in oleic acid at concentrations as high as 100 μM (the solubility limit of BPE in oleic acid). To further justify the versatile applicability of our technique, additional measurement with adenine was carried out. In Fig. 5c , unique Raman transition of adenine is clearly observed around 730 cm −1 . 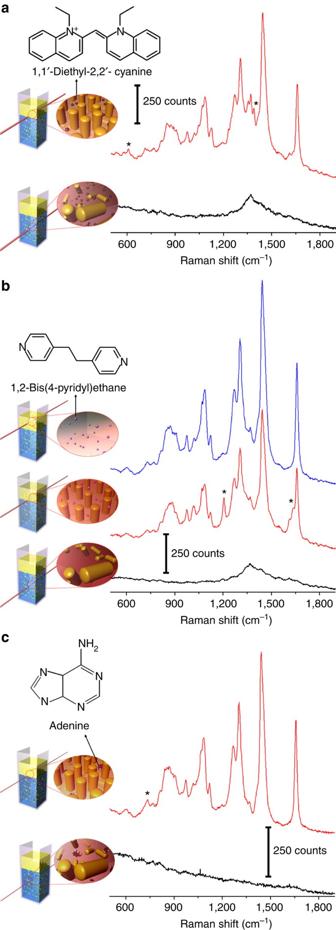Figure 5: Versatility of the interfacial liquid-state SERS technique. (a) SERS signals of aqueous 10 μM DCI solutions at the oleic acid–water interface (top) and within the water layer (bottom). (b) SERS signals of 10 μM BPE in oleic acid within the oleic acid layer (top), at the oleic acid–water interface (middle) and within the water layer (bottom). (c) SERS signals of 1 μM adenine at the oleic acid–water interface (top) and within the water layer (bottom). Positions marked with an asterisk indicate representative Raman peaks of DCI, BPE and adenine (see alsoSupplementary Fig. S15). Figure 5: Versatility of the interfacial liquid-state SERS technique. ( a ) SERS signals of aqueous 10 μM DCI solutions at the oleic acid–water interface (top) and within the water layer (bottom). ( b ) SERS signals of 10 μM BPE in oleic acid within the oleic acid layer (top), at the oleic acid–water interface (middle) and within the water layer (bottom). ( c ) SERS signals of 1 μM adenine at the oleic acid–water interface (top) and within the water layer (bottom). Positions marked with an asterisk indicate representative Raman peaks of DCI, BPE and adenine (see also Supplementary Fig. S15 ). Full size image In summary, we have demonstrated a versatile liquid–liquid interface capable of functioning as a substrate for the orientation of colloidal GNRs. The observed self-orientation allowed for the development of a substrate-free liquid-state SERS technique. The vertical orientation of the GNRs in a stable trapping mode is directly visualized by dark-field scattering imaging, which is further supported by Raman experiments. According to our calculations, interfacial energy is minimized when the GNRs adopt a vertical orientation at the oleic acid–water interface. Spontaneous vertical alignment of GNRs results in the significant additional enhancement of SERS signals by up to three to four orders of magnitude higher than those measured directly from solutions containing randomly oriented GNRs. Self-oriented GNRs at the oil–water interface are also capable of probing oil-soluble molecules. Our technique is simple-to-use and easy-to-follow as it consists of mixing a solution of GNRs with targets of interest, adding oleic acid, shining a light at the clearly visible interface and collecting fingerprint information. We anticipate that our finding of the self-orientation of GNRs at the liquid interface and a versatile interfacial liquid-state SERS technique (1) significantly expands the flexibility of SERS, (2) opens a new avenue for high-throughput screening of biologically and environmentally important molecules and the precise characterization of soft matters, and (3) provides a new route to the formation of functional materials. Materials All chemicals, including R6G, DCI, BPE, adenine and oleic acid were purchased from Sigma Aldrich Inc. and used as received. Preparation and characterization of GNRs Before synthesis, all glassware was treated with piranha solution (H 2 SO 4 :H 2 O 2 =7:3 v/v , warning: this solution is highly acidic and a strong oxidant) for 30 min, and then rinsed with copious amounts of deionized water. GNRs were synthesized by a previously reported method [23] . GNRs were prepared by a seed-mediated growth method, which progresses from small spherical gold seeds (~4 nm) and a weak reducing agent (ascorbic acid) in the presence of a directing surfactant (CTAB) for the subsequent reduction of gold ions on the seed. In detail, 47.5 ml of 0.1 M CTAB was mixed 425 μl of 0.01 M silver nitrate aqueous solution, 2.5 ml of 0.01 M HAuCl 4 trihydrate (aq) and 275 μl of 0.10 M ascorbic acid (aq), respectively, with continuous stirring. Sixty microlitre of the seed solution was finally injected into the mixture to initiate the growth of GNRs. The aspect ratio of GNRs was controlled by simply varying the amount of silver ion present in the solution. The shape and optical properties of the synthesized GNRs were characterized by transmission electron microscopy (TEM) and ultraviolet–vis spectroscopy. TEM samples were prepared by carefully dropping 10 μl of the dispersion onto a carbon-coated 300 mesh TEM grid (Ted Pella Inc.). Dark-field scattering imaging For the dark-field imaging, a Zeiss inverted microscope equipped with a dark-field water immersion condenser (NA=1.2~1.4) [36] , [37] and a DSLR camera (Canon Mark 5D II) was used. A home-made PDMS fluidic chamber was prepared. During GNR trapping, movie was recorded in real-time ( Supplementary Movies 2 and 3 ). Brownian motion of GNRs in water unlike a stable trapping mode of GNRs at the interface was also recorded ( Supplementary Movie 4 ). A linear polarizer (Thorlabs part # LPVIS050) was installed and rotated at the light entrance of the dark-field condenser to characterize the orientation of GNRs at the interface. In order to characterize the motion and orientation of individual GNRs trapped at the interface, GNR concentration was properly diluted. It is difficult to resolve individual scattering spots at the interface owing to the strong background scattering from GNRs in a solution unless the GNR solution is diluted ( Supplementary Fig. S17 ). Raman and SERS measurement A commercial Raman spectrometer QE65000 (Ocean Optics Inc.) and 785-nm laser module I0785MM0350MS (Innovative Photonic Solution Inc.) was used for Raman and SERS measurements. The illumination source was a 785 nm laser operated at a power of 250 mW and an integration time of 100 ms was employed in the Raman measurements. Measurements were performed over a wavenumber range of 200 to 2,250 cm −1 . In a typical interfacial liquid-state SERS experiment, 1 ml of freshly made GNR solution and 250 μl of target molecule were introduced into a cuvette. The mixture was diluted by 1.25 ml of deionized water. Following preparation of the mixture of GNRs and target molecules, 500 μl of oleic acid was introduced to form the oleic acid–water interface. We fixed the laser position with the information of z axis position (that is, height) of oleic acid–water interface and the focal length of the laser. The z axis position was calculated from the volume ratio of oleic acid and water. In addition, the laser was positioned at the same xy plane of the oleic acid–water interface. The x (or y )-axis position (that is, horizontal distance) between the laser and the oleic acid–water interface was equal to the focal length of the laser. All SERS data were collected within 20 s following the addition of oleic acid in order to neglect the effects of any diffusion factors (for example, diffusion of GNRs and target molecules to the interface) on the experiments. The illumination source was a 785 nm laser operated at a power of 250 mW and an integration time of 3 s was employed in the SERS experiments. Note that ethanol-driven assembly of GNRs at the oleic acid–water interface was possible and, however, no SERS signal from such assembly was observed ( Supplementary Fig. S18 ). SERS signals were remarkably decreased under strong acidic and basic conditions ( Supplementary Fig. S19 ). Calculation of an interfacial energy We analytically derived equations for the surface area of GNR exposed to each medium. Then, interfacial energy ( E ) for the specific orientation and position was numerically calculated based on the equation (1). The detailed explanation for calculation of interfacial energy is included in the Supplementary Note 1 and the general assumptions for the calculation of interfacial energy by using equation (1) are also included in the Supplementary Note 2 . How to cite this article: Kim K. et al. Interfacial liquid-state surface-enhanced Raman spectroscopy. Nat. Commun. 4:2182 doi: 10.1038/ncomms3182 (2013).